Generation of colonic IgA-secreting cells in the caecal patch Gut-associated lymphoid tissues are responsible for the generation of IgA-secreting cells. However, the function of the caecal patch, a lymphoid tissue in the appendix, remains unknown. Here we analyse the role of the caecal patch using germ-free mice colonized with intestinal bacteria after appendectomy. Appendectomized mice show delayed accumulation of IgA + cells in the large intestine, but not the small intestine, after colonization. Decreased colonic IgA + cells correlate with altered faecal microbiota composition. Experiments using photoconvertible Kaede-expressing mice or adoptive transfer show that the caecal patch IgA + cells migrate to the large and small intestines, whereas Peyer’s patch cells are preferentially recruited to the small intestine. IgA + cells in the caecal patch express higher levels of CCR10. Dendritic cells in the caecal patch, but not Peyer’s patches, induce CCR10 on cocultured B cells. Thus, the caecal patch is a major site for generation of IgA-secreting cells that migrate to the large intestine. Intestinal lamina propria plasma cells secrete IgA as a dimer, which is transported to the intestinal lumen by polymeric immunoglobulin receptor [1] , [2] , [3] , [4] . In the intestinal lumen, secretory IgA binds pathogens and pathogen-derived antigens to limit their invasion into the body [5] , [6] . In addition, secretory IgA contributes to the maintenance of gut homeostasis by regulating the activities and compositions of commensal bacteria [5] , [7] , [8] , [9] . Dysregulation of gut homeostasis caused by defective IgA responses can compromise host defenses against intestinal pathogenic bacteria and correlates with autoimmune diseases [10] , [11] , [12] . IgA-secreting cells develop in gut-associated lymphoid tissues (GALTs) such as Peyer’s patches and solitary intestinal lymphoid tissues (SILTs) including cryptopatches, colonic patches and isolated lymphoid follicles (ILFs). Peyer’s patches and ILF contribute to generation of IgA-secreting cells by different mechanisms [2] , [13] , [14] . However, it still remains unclear where and how IgA acquires antigen specificities and diversities. So far, characterization of IgA has focused on plasma cells residing in the small intestine. It has recently been reported that IgAs derived from the small and large intestines have differential repertoires [15] . It has also been reported that CCR9 mediates migration of IgA-secreting cells to the small intestine but not the large intestine [16] , whereas CCR10 is involved in migration to both the small and large intestines [17] . However, it remains unclear where IgA-secreting plasma cells that migrate to the large intestine are generated. In the appendix, a blind-ended tract linking the caecum, are lymphoid clusters called caecal patches. Compared with human caecal patches, which are present as multiple small clusters, mice possess a single large lymphoid cluster in the appendix [18] . As with Peyer’s patches, caecal patches are covered by a monolayer of epithelial cells, among which M cells are present. Antigen-specific immunoglobulin responses and immunoglobulin diversification have been reported to occur in the appendix of rabbits [19] , [20] . Contrary to the above-mentioned evidences indicating that caecal patches are related to Peyer’s patches, electron microscopy analysis has indicated that M cells on caecal patches have differential morphology to those on Peyer’s patches [21] . Furthermore, it has been reported that appendectomy ameliorates intestinal inflammation observed in Tcra −/− mice or dextran sodium sulphate-treated mice [18] , [22] . Thus, caecal patches in the appendix are thought to possess unique functions compared with other GALTs. However, the roles of caecal patches in mucosal immune responses remain unclear. In this study, we analysed the function of the mouse caecal patch using germ-free mice, in which intestinal IgA-secreting cells are severely decreased because of the absence of commensal bacteria. Surgical resection of the appendix results in slower accumulation of IgA-secreting cells in the large intestine, but not the small intestine, after conventionalization of germ-free mice. IgA + cells in the caecal patch migrate to both the large and small intestines, whereas those in Peyer’s patches are preferentially recruited to the small intestine. IgA + cells generated in the caecal patch express increased levels of CCR10 compared with cells in Peyer’s patches. Decreased number of colonic IgA-secreting cells correlates with altered composition of faecal microbiota in appendectomized mice at the early time point after colonization. These findings suggest that the caecal patch is a major site for the generation of IgA-secreting cells that migrate to the large intestine. Similar characteristics of caecal patches and Peyer’s patches There exists a single lymphoid cell cluster in the appendix of mice called caecal patch [18] ( Fig. 1a ). We compared immunological aspects of the characteristics of the caecal patch and Peyer’s patches by immunohistochemistry ( Fig. 1b ). The caecal patch showed similar patterns of expression of CD4, B220 and CD11c to Peyer’s patches, which are composed of B-cell-rich follicles, T-cell-rich parafollicular areas and a CD11c + cell-rich subepithelial dome region. Flow cytometry analysis indicated that the caecal patch and Peyer’s patches contained similar numbers of IgM + B cells, IgA + B cells, CD4 + cells and CD11c + cells ( Fig. 1c , Supplementary Fig. 1 ). In addition, mRNA expression of genes encoding APRIL, BAFF and AID, which are involved in the class switching of immunoglobulin, in the caecal patch was equivalent to that observed in Peyer’s patches and mesenteric lymph nodes ( Fig. 1d ). Peyer’s patches in germ-free mice have been reported to be small [23] . Similarly, the size of the caecal patch in germ-free mice was reduced compared with specific-pathogen-free mice, indicating that the development of the caecal patch is dependent on commensal microbiota ( Fig. 1e ). Organogenesis of Peyer’s patches has been reported to be initiated by the interaction of haematopoietic Rorγt + lymphoid tissue inducer (LTi) cells and stromal cells, which receive lymphotoxin signalling from LTi cells via lymphotoxin β receptor (LTβR). Mice lacking Rorγt( Rorc ( gt ) gfp/gfp mice) showed impaired development of LTi cells, and accordingly lacked Peyer’s patches [24] . aly / aly mice that had a mutated gene encoding NF-κB-inducing kinase (NIK), which mediates LTβR signalling, showed impaired development of Peyer’s patches [25] . These mutant mice also showed impaired caecal patch development ( Fig. 1f ). As previously reported, Peyer’s patch cells from T-cell-deficient ( Tcrb −/− Tcrd −/− ) mice produced lower, but substantial, amounts of IgA than those of the wild-type mice [26] , [27] , [28] ( Fig. 1g ). IgA production from caecal patch cells of Tcrb −/− Tcrd −/− mice was also similarly reduced, thus indicating that the caecal patch as well as Peyer’s patches mediate both T cell-dependent and -independent IgA inductions. Thus, the caecal patch and Peyer’s patches show analogous features of immunological structures, function and developmental processes. 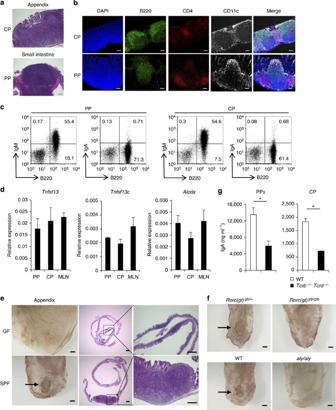Figure 1: Similar immunological characteristics of the caecal patch and Peyer’s patches. (a) Haematoxylin and eosin staining of the caecal patch (CP) in the appendix and Peyer’s patches (PP) in the small intestine of specific-pathogen-free mice. Scale bars, 100 μm. (b) Distribution of immune cells in CP and PP. Frozen sections were stained for B220 (green), CD4 (red), CD11c (grey) and DAPI (blue), and analysed by confocal fluorescence microscopy. Scale bars, 100 μm. (c) B-cell populations in CP and PP of specific-pathogen-free (SPF) mice. Cells were stained with anti-IgA, IgM and B220 mAbs, and analysed by flow cytometry. Numbers within dot plots indicate percentages of cells in respective areas. (d) Expression of immunoglobulin class switching-related genes. Expression of mRNA forTnfsf13(encoding APRIL),Tnfsf13c(encoding BAFF) andAicda(encoding AID) in PP, CP and mesenteric lymph node (MLN) were quantitatively analysed by real-time RT-PCR, and normalized to that ofGapdh. Data represent mean±s.d. (n=4 per group), and representations of two independent experiments are shown. (e) Development of the caecal patch in SPF or germ-free (GF) mice. Left: gross appearance of the appendix. The caecal patch was visualized based on a B220+cluster of whole-mount staining. Middle and right: haematoxylin and eosin staining of the appendix. The boxed areas in the middle panels are enlarged on the right. Scale bars, 1 mm (left), 300 μm (middle) and 100 μm (right). (f) Development of the caecal patch inRorc(gt)gfp/+orRorc(gt)gfp/gfpmice (upper) and WT oraly/alymice (lower). Arrows indicate CP (e,f). Original magnification, × 7 (left panels ineandf). Scale bars, 1 mm. (g) IgA production by mononuclear cells from PP and CP. Mononuclear cells from PP and CP of WT andTcrb−/−Tcrd−/−mice were cultured for 3 days and the supernatant was analysed by ELISA. Data represent mean±s.d. of triplicate samples in one experiment, and representations of two independent experiments are shown. Statistical analyses were performed with the Student’st-test. *P<0.05. Figure 1: Similar immunological characteristics of the caecal patch and Peyer’s patches. ( a ) Haematoxylin and eosin staining of the caecal patch (CP) in the appendix and Peyer’s patches (PP) in the small intestine of specific-pathogen-free mice. Scale bars, 100 μm. ( b ) Distribution of immune cells in CP and PP. Frozen sections were stained for B220 (green), CD4 (red), CD11c (grey) and DAPI (blue), and analysed by confocal fluorescence microscopy. Scale bars, 100 μm. ( c ) B-cell populations in CP and PP of specific-pathogen-free (SPF) mice. Cells were stained with anti-IgA, IgM and B220 mAbs, and analysed by flow cytometry. Numbers within dot plots indicate percentages of cells in respective areas. ( d ) Expression of immunoglobulin class switching-related genes. Expression of mRNA for Tnfsf13 (encoding APRIL), Tnfsf13c (encoding BAFF) and Aicda (encoding AID) in PP, CP and mesenteric lymph node (MLN) were quantitatively analysed by real-time RT-PCR, and normalized to that of Gapdh . Data represent mean±s.d. ( n =4 per group), and representations of two independent experiments are shown. ( e ) Development of the caecal patch in SPF or germ-free (GF) mice. Left: gross appearance of the appendix. The caecal patch was visualized based on a B220 + cluster of whole-mount staining. Middle and right: haematoxylin and eosin staining of the appendix. The boxed areas in the middle panels are enlarged on the right. Scale bars, 1 mm (left), 300 μm (middle) and 100 μm (right). ( f ) Development of the caecal patch in Rorc(gt) gfp/+ or Rorc ( gt ) gfp/gfp mice (upper) and WT or aly/aly mice (lower). Arrows indicate CP ( e , f ). Original magnification, × 7 (left panels in e and f ). Scale bars, 1 mm. ( g ) IgA production by mononuclear cells from PP and CP. Mononuclear cells from PP and CP of WT and Tcrb −/− Tcrd −/− mice were cultured for 3 days and the supernatant was analysed by ELISA. Data represent mean±s.d. of triplicate samples in one experiment, and representations of two independent experiments are shown. Statistical analyses were performed with the Student’s t -test. * P <0.05. Full size image Delayed colonic IgA + cell recruitment without caecal patch Given that the caecal patch showed similar properties to Peyer’s patches, which are typical GALTs mediating immune responses, we investigated the immunological function of the caecal patch by generating caecal patch-deficient mice. To assess the effect of caecal patch deficiency on the development of intestinal immunity, we utilized germ-free mice, which showed normal development of the adaptive immune system after bacterial colonization in the gut. We removed the appendix of germ-free mice by surgery, and then transferred and reared them in a conventionalized (specific-pathogen-free) environment ( Supplementary Fig. 2 ). At 4 weeks after conventionalization, mice were analysed for the number of IFN-γ-, IL-17- and IL-10-producing CD4 + T cells and IgA + cells in the small and large intestines ( Fig. 2a,b and Supplementary Fig. 3 ). IFN-γ-, IL-17- and IL-10-producing CD4 + T cells all increased in numbers similarly in the small and large intestines of sham-operated and appendectomized mice. IgA + cells in the small intestine of sham-operated and appendectomized mice also increased to a similar extent after conventionalization. However, the number of IgA + cells in the large intestine markedly decreased in appendectomized mice compared with sham-operated mice. The decrease in number of IgA + cells in large intestinal lamina propria was further confirmed by immunohistochemical analysis ( Fig. 2c ). IgA + cells were scarcely observed in germ-free mice, and conventionalization of sham-operated germ-free mice increased the number of IgA + cells. In contrast, the number of IgA + cells in large intestinal lamina propria did not dramatically increase after conventionalization of germ-free mice with the appendectomy at 4 weeks after conventionalization. We next analysed concentration of secretory IgA in faeces and serum at 4 weeks after conventionalization ( Fig. 2d ). Levels of secretory IgA in faeces, but not in serum, in appendectomized mice were lower than those in sham-operated mice. Thus, accumulation of IgA-secreting cells selectively decreased in the large intestine of appendectomized mice at 4 weeks after conventionalization. We then analysed time-dependent increase of IgA + cells in the large intestine by measuring IgA + cell number at 2, 4 and 8 weeks after conventionalization ( Fig. 3a–c ). At 2 weeks as well as 4 weeks, the number of IgA + cells was markedly decreased in appendectomized mice. However, at 8 weeks, the number of IgA + cells of appendectomized mice was comparable to that of sham-operated mice. Taken together, these findings indicate that accumulation of IgA-secreting cells to the large intestine was delayed in mice with appendectomy. 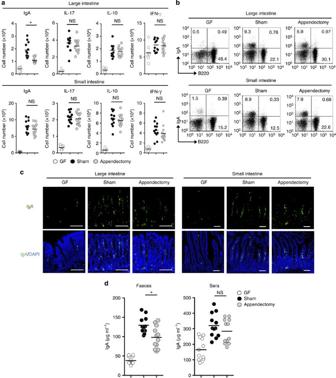Figure 2: Decreased IgA-secreting cells in large intestinal lamina propria of appendectomized germ-free mice after conventionalization. (a,b) Lamina propria lymphocytes were isolated from appendectomized or sham-operated germ-free(GF) mice at 4 weeks after conventionalization, and stained for surface IgA/B220 or intracellular IL-17/IFN-γ/IL-10 in CD4+population. (a) Total numbers of IgA+B220−cells as well as IL-17-, IFN-γ- and IL-10-positive CD4+cells in the large (upper) and the small intestine (lower) are shown. Each symbol represents an individual mouse, and horizontal bars indicate the mean. (b) Representative dot plots for cells stained with anti-IgA and B220 of appendectomized and sham-operated mice. Numbers within plots indicate percentages of cells in respective areas. (c) Distribution of IgA+cells in the small and large intestines. Frozen sections were stained with anti-IgA mAb (green) and DAPI (blue). Scale bars, 100 μm. (d) Faeces and sera were collected from appendectomized (n=12) or sham-operated mice (n=12) at 4 weeks after conventionalization and GF mice (n=12), and IgA levels of faeces and sera were determined by ELISA. Each symbol represents an individual mouse, and horizontal bars indicate the mean. Statistical analyses were performed with the Student’st-test. *P<0.05. NS, not significant. Figure 2: Decreased IgA-secreting cells in large intestinal lamina propria of appendectomized germ-free mice after conventionalization. ( a , b ) Lamina propria lymphocytes were isolated from appendectomized or sham-operated germ-free(GF) mice at 4 weeks after conventionalization, and stained for surface IgA/B220 or intracellular IL-17/IFN-γ/IL-10 in CD4 + population. ( a ) Total numbers of IgA + B220 − cells as well as IL-17-, IFN-γ- and IL-10-positive CD4 + cells in the large (upper) and the small intestine (lower) are shown. Each symbol represents an individual mouse, and horizontal bars indicate the mean. ( b ) Representative dot plots for cells stained with anti-IgA and B220 of appendectomized and sham-operated mice. Numbers within plots indicate percentages of cells in respective areas. ( c ) Distribution of IgA + cells in the small and large intestines. Frozen sections were stained with anti-IgA mAb (green) and DAPI (blue). Scale bars, 100 μm. ( d ) Faeces and sera were collected from appendectomized ( n =12) or sham-operated mice ( n =12) at 4 weeks after conventionalization and GF mice ( n =12), and IgA levels of faeces and sera were determined by ELISA. Each symbol represents an individual mouse, and horizontal bars indicate the mean. Statistical analyses were performed with the Student’s t -test. * P <0.05. NS, not significant. 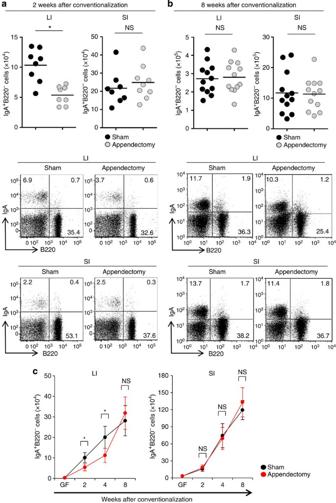Figure 3: The number of IgA-secreting cells in the large intestine at 2 and 8 weeks after conventionalization. (a,b) Lamina propria lymphocytes were prepared from appendectomized or sham-operated mice at 2 weeks (a) and 8 weeks (b) after conventionalization, and analysed for the expression of surface IgA and B220 by flow cytometry. Total numbers of IgA+B220−cells in the small or large intestines are shown. Each symbol represents an individual mouse, and horizontal bars indicate the mean. Representative dot plots of intestinal leukocytes prepared from appendectomized and sham-operated mice are shown. Numbers within plots indicate percentages of cells in respective areas. (c) The numbers of IgA+B220−cells in the small and large intestines of appendectomized and sham-operated mice at indicated time points after conventionalization. The experiments were performed more than two times with similar results. Data represent mean±s.d. (four mice per group). SI, small intestine; LI, large intestine. Statistical analyses were performed with the Student’st-test. *P<0.05. NS: not significant. Full size image Figure 3: The number of IgA-secreting cells in the large intestine at 2 and 8 weeks after conventionalization. ( a , b ) Lamina propria lymphocytes were prepared from appendectomized or sham-operated mice at 2 weeks ( a ) and 8 weeks ( b ) after conventionalization, and analysed for the expression of surface IgA and B220 by flow cytometry. Total numbers of IgA + B220 − cells in the small or large intestines are shown. Each symbol represents an individual mouse, and horizontal bars indicate the mean. Representative dot plots of intestinal leukocytes prepared from appendectomized and sham-operated mice are shown. Numbers within plots indicate percentages of cells in respective areas. ( c ) The numbers of IgA + B220 − cells in the small and large intestines of appendectomized and sham-operated mice at indicated time points after conventionalization. The experiments were performed more than two times with similar results. Data represent mean±s.d. (four mice per group). SI, small intestine; LI, large intestine. Statistical analyses were performed with the Student’s t -test. * P <0.05. NS: not significant. Full size image Altered faecal microbiota composition in appendectomized mice As secretory IgA is responsible for the control of intestinal bacteria, we analysed the composition of faecal microbiota in appendectomized and sham-operated mice at 4 weeks after conventionalization by pyrosequence-based 16S rRNA gene profiling. The rarefaction curve showed that the estimated operational taxonomic units (OTUs) of appendectomized mice were less abundant than those of sham-operated mice and that the sufficient sequencing depth has been achieved in both groups ( Fig. 4a ). In the class distribution, the relative abundance of several bacterial groups such as Bacilli , Erysipelotrichi and Gammaproteobacteria in appendectomized mice was higher than that in sham-operated mice; Mollicutes , Deferribacteres , Betaproteobacteria and Deltaproteobacteria were less abundant in appendectomized mice ( Fig. 4b , Supplementary Table 1 ). Analyses at the other levels also showed that the relative abundance of many bacterial groups was significantly different between appendectomized and sham-operated groups ( Supplementary Fig. 4a–c , Supplementary Tables 2–4 ). Principal coordinate analysis using the relative abundance of OTUs indicated that bacterial community of appendectomized mice was clearly separated from that of sham-operated mice at 4 weeks after conventionalization ( Fig. 4c , Supplementary Data 1 ). We then analysed faecal microbiota composition in appendectomized mice at 8 weeks after conventionalization when colonic IgA-secreting cells were normalized. Bacterial community of appendectomized mice at 8 weeks after conventionalization was similar to that of sham-operated mice ( Fig. 4d,e ). Thus, at 4 weeks after conventionalization, microbiota composition was altered in mice with appendectomy, but in accordance with normalized numbers of colonic IgA-secreting cells at 8 weeks, the alteration of faecal microbiota composition disappeared. 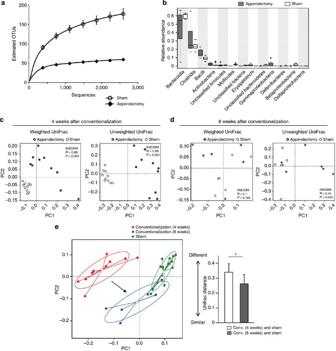Figure 4: Altered composition of faecal microbiota in appendectomized mice. Faecal microbiota in mice with appendectomy (n=10) and sham-surgery (n=10) at 4 weeks and 8 weeks after conventionalization was analysed by pyrosequence-based 16S rRNA gene profiling. (a) Rarefaction curves of sham-operated and appendectomized groups at 4 weeks after conventionalization. The vertical axis shows the number of observed species that would be expected to be found after sampling the number of sequences shown on the horizontal axis. The number of taxa was at a 3% dissimilarity level. Data represent mean±s.d. (b) A box plot of class level-bacterial composition of appendectomized and sham-operated mice at 4 weeks after conventionalization. The box for each group represents the interquartile range (25–75th percentile) and the line within the box is the median value. The bottom and top bars indicate the 10th and 90th percentile, respectively. Open circles represent outlier values. The results of statistical test were described inSupplementary Table 1. (c,d) The principal coordinate analysis (PCoA) using OTUs based on the weighted (left) and unweighted (right) UniFrac distances. Faecal microbiota of appendectomized mice at 4 weeks (c) or 8 weeks (d) after conventionalization was compared with that of sham-operated mice. For statistical analysis, ANOSIM was calculated using R package ‘Vegan’. (e) PCoA of faecal microbiota in mice with appendectomy and sham-surgery at 4 weeks and 8 weeks after conventionalization using OTUs (left). Red, blue and green circles indicate the clusters of mice with appendectomy at 4 weeks, 8 weeks after conventionalization and sham-operated mice, respectively. The UniFrac distance is calculated between pairs of samples (right). Statistical analyses were performed with the Student’st-test. *P<0.05. Figure 4: Altered composition of faecal microbiota in appendectomized mice. Faecal microbiota in mice with appendectomy ( n =10) and sham-surgery ( n =10) at 4 weeks and 8 weeks after conventionalization was analysed by pyrosequence-based 16S rRNA gene profiling. ( a ) Rarefaction curves of sham-operated and appendectomized groups at 4 weeks after conventionalization. The vertical axis shows the number of observed species that would be expected to be found after sampling the number of sequences shown on the horizontal axis. The number of taxa was at a 3% dissimilarity level. Data represent mean±s.d. ( b ) A box plot of class level-bacterial composition of appendectomized and sham-operated mice at 4 weeks after conventionalization. The box for each group represents the interquartile range (25–75th percentile) and the line within the box is the median value. The bottom and top bars indicate the 10th and 90th percentile, respectively. Open circles represent outlier values. The results of statistical test were described in Supplementary Table 1 . ( c , d ) The principal coordinate analysis (PCoA) using OTUs based on the weighted (left) and unweighted (right) UniFrac distances. Faecal microbiota of appendectomized mice at 4 weeks ( c ) or 8 weeks ( d ) after conventionalization was compared with that of sham-operated mice. For statistical analysis, ANOSIM was calculated using R package ‘Vegan’. ( e ) PCoA of faecal microbiota in mice with appendectomy and sham-surgery at 4 weeks and 8 weeks after conventionalization using OTUs (left). Red, blue and green circles indicate the clusters of mice with appendectomy at 4 weeks, 8 weeks after conventionalization and sham-operated mice, respectively. The UniFrac distance is calculated between pairs of samples (right). Statistical analyses were performed with the Student’s t -test. * P <0.05. Full size image To exclude the possibility that the incision of the appendix itself caused the slow accumulation of IgA-secreting cells and the altered composition of microbiota in the large intestine, we cut and sutured the appendix without excision, and analysed the number of IgA-secreting cells and faecal microbiota at 4 weeks after conventionalization ( Supplementary Fig. 5a–d ). In these enterotomized mice, no alteration of the IgA-secreting cells and microbiota composition was observed compared with sham-operated mice, which underwent incision of the abdomen alone. Thus, appendectomized mice, which showed delayed accumulation of IgA + cells in the large intestine, had altered configurations of faecal microbiota at 4 weeks after conventionalization. Recruitment of caecal patch IgA + cells to the colon We analysed the mechanisms for the slower increase of colonic IgA-secreting cells in appendectomized mice using Kaede-transgenic mice, in which in vivo cell migration can be monitored [29] . Kaede is a photoconvertible protein, changing fluorescence from green to red with exposure of violet light. We generated Kaede bone marrow chimeric mice, in which bone marrow cells were reconstituted with those of Kaede-transgenic mice. The caecal patch from Kaede bone marrow chimeric mice was exposed to violet light for 5 min to induce photoconversion of Kaede proteins expressed in haematopoietic cell types present in this region. After exposure, 93.8±3.2% of cells isolated from caecal patches expressed a red fluorescence signal (Kaede-red) ( Supplementary Fig. 6 ). At 3 and 7 days after photoconversion, the number of Kaede-red cells gradually decreased in the caecal patch ( Fig. 5a ). Accordingly, Kaede-red IgA + B220 − cells increased similarly in the lamina propria of the small and large intestines at the 7-day time point ( Fig. 5b ). We also exposed Peyer’s patches to violet light, and analysed migration of Peyer’s patch-derived IgA + cells to intestinal lamina propria. Kaede-red IgA + B220 − cells were observed both in the small and large intestines at 7 days after photoconversion. However, the percentage of Kaede-red IgA + cells in total IgA + cells was markedly reduced in the large intestine compared with the small intestine ( Fig. 5c ). These findings indicate that IgA-secreting cells generated in the caecal patch migrate to both the small and large intestines, but IgA-secreting cells generated in Peyer’s patches preferentially migrate to the small intestine. To corroborate these findings, we transferred CD45.2 + B220 + cells from caecal patches and Peyer’s patches into CD45.1 + mice. At 7 days after transfer, CD45.2 + IgA + cells in the small and large intestines of CD45.1 + mice were measured ( Fig. 5d ). Similarly to the results obtained from experiments using Kaede bone marrow chimeric mice, IgA + cells isolated from caecal patches migrated to both the small and large intestines. In contrast, IgA + cells isolated from Peyer’s patches were preferentially recruited to the small intestine. Taken together, these findings suggest that IgA-secreting cells generated in Peyer’s patches mainly migrate to the small intestine, whereas IgA-secreting cells generated in the caecal patch are programmed to be recruited to both the small and large intestines. In accordance with these findings, the caecum/appendix showed a similar pattern of bacterial composition to the large intestine rather than the small intestine ( Supplementary Figs 7 and 8 ), indicating that large intestine-types of intestinal bacteria residing in the caecum/appendix may contribute to the generation of IgA that acts on bacteria of the large intestine. 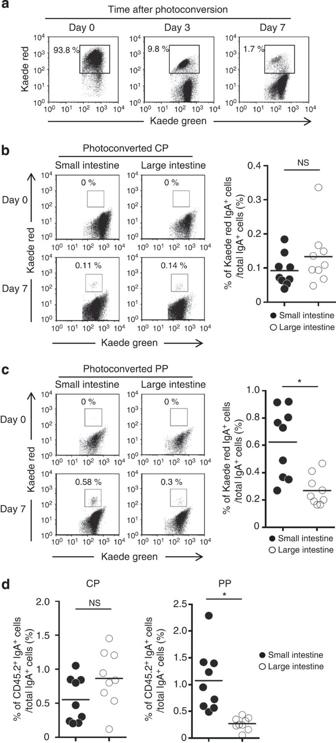Figure 5: Recruitment of caecal patch, but not Peyer’s patch, IgA-secreting cells to the colon. (a) The caecal patch in the appendix from Kaede bone marrow chimeric mice were exposed to violet light for 5 min and resected immediately (day 0), or 3 and 7 days after violet light exposure. Cells from photoconverted caecal patches were subjected to flow cytometry at indicated time points to evaluate photoconversion. Numbers within plots indicate percentages of cells in respective areas. Data are representative of three independent experiments. (b,c) The caecal patch (CP) (b) or Peyer’s patches (PP) (c) were exposed to violet light for 5 min, and the percentages of Kaede-red IgA+cells in total IgA+cells in the intestines were analysed at 7 days after photoconversion. Representative dot plots of cells in the intestinal lamina propria are shown (left). Right panel shows the percentages of photoconverted IgA+cells in total IgA+cells of intestinal lamina propria. Each symbol represents an individual mouse, and horizontal bars indicate the mean. (d) B220+cells from CD45.2 mice were transferred into CD45.1 C57BL/6 recipient mice. CD45.2+IgA+cells in intestinal lamina propria from CD45.1 C57BL/6 mice were analysed at 7 days after cell transfer. Data show the percentages of CD45.2+IgA+cells in total IgA+cells of intestinal lamina propria. Each symbol represents an individual mouse, and horizontal bars indicate the mean. Statistical analyses were performed with the Student’st-test. *P<0.05. NS, not significant. Figure 5: Recruitment of caecal patch, but not Peyer’s patch, IgA-secreting cells to the colon. ( a ) The caecal patch in the appendix from Kaede bone marrow chimeric mice were exposed to violet light for 5 min and resected immediately (day 0), or 3 and 7 days after violet light exposure. Cells from photoconverted caecal patches were subjected to flow cytometry at indicated time points to evaluate photoconversion. Numbers within plots indicate percentages of cells in respective areas. Data are representative of three independent experiments. ( b , c ) The caecal patch (CP) ( b ) or Peyer’s patches (PP) ( c ) were exposed to violet light for 5 min, and the percentages of Kaede-red IgA + cells in total IgA + cells in the intestines were analysed at 7 days after photoconversion. Representative dot plots of cells in the intestinal lamina propria are shown (left). Right panel shows the percentages of photoconverted IgA + cells in total IgA + cells of intestinal lamina propria. Each symbol represents an individual mouse, and horizontal bars indicate the mean. ( d ) B220 + cells from CD45.2 mice were transferred into CD45.1 C57BL/6 recipient mice. CD45.2 + IgA + cells in intestinal lamina propria from CD45.1 C57BL/6 mice were analysed at 7 days after cell transfer. Data show the percentages of CD45.2 + IgA + cells in total IgA + cells of intestinal lamina propria. Each symbol represents an individual mouse, and horizontal bars indicate the mean. Statistical analyses were performed with the Student’s t -test. * P <0.05. NS, not significant. Full size image Enhanced CCR10 expression in caecal patch IgA + cells It has been reported that CCR9 and CCR10 mediate the migration of IgA + cells to the intestinal lamina propria [30] . Therefore, we used anti-CCR9 mAb and CCL27-Fc chimera protein to analyse surface expression of CCR9 and CCR10 on IgA + cells, which were positive for the plasmablast marker CD138 ( Supplementary Fig. 9 ), in the caecal patch and Peyer’s patch ( Fig. 6a,b ). CCR9 was similarly expressed on IgA + cells in the caecal patch and Peyer’s patch. In contrast, expression of CCR10 determined by CCL27-binding in caecal patch IgA + cells was markedly higher than IgA + cells in Peyer’s patches. 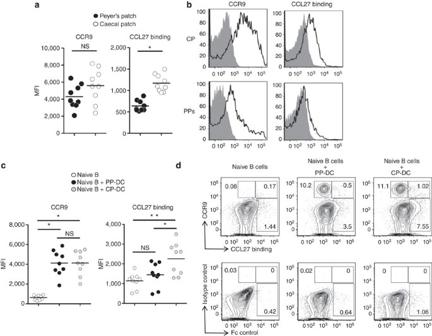Figure 6: Enhanced CCR10 expression in caecal patch IgA-producing cells. (a,b) Expression of CCR9 and CCR10 on IgA+cells in Peyer’s patch and the caecal patch. IgA+B220+cells prepared from Peyer’s patches (PP) or caecal patch (CP) of specific-pathogen-free mice were analysed for expression of CCR9 and CCR10 using anti-CCR9 mAb and CCL27-Fc chimera protein, respectively. (a) The mean fluorescence intensity (MFI) of the indicated surface markers on PP or CP IgA+cells is shown. Each symbol represents an individual mouse, and horizontal bars indicate the mean. (b) Histograms gated on IgA+B220+cells from PP or CP. Solid line: CCR9 expression or CCL27 binding, grey histogram: human IgG Fc or isotype control. (c,d) Induction of CCR9 and CCR10 on IgA+cells by GALT-DCs. CD11c+cells were isolated from PP and CP of mice injected with B16 melanoma cells secreting Flt3L. Splenic naive B cells were cultured in the presence of antibody to IgM alone or with CP-derived DCs (CP-DC) or PP-derived DCs (PP-DC). After 4 days, B cells were analysed for CCR9 expression and CCL27 binding. (c) Each symbol represents an individual mouse, and horizontal bars indicate the mean. (d) Representative dot blots gated on B220+cells are shown. Statistical analyses were performed with the Student’st-test. *P<0.05. **P<0.005, NS, not significant. Figure 6: Enhanced CCR10 expression in caecal patch IgA-producing cells. ( a , b ) Expression of CCR9 and CCR10 on IgA + cells in Peyer’s patch and the caecal patch. IgA + B220 + cells prepared from Peyer’s patches (PP) or caecal patch (CP) of specific-pathogen-free mice were analysed for expression of CCR9 and CCR10 using anti-CCR9 mAb and CCL27-Fc chimera protein, respectively. ( a ) The mean fluorescence intensity (MFI) of the indicated surface markers on PP or CP IgA + cells is shown. Each symbol represents an individual mouse, and horizontal bars indicate the mean. ( b ) Histograms gated on IgA + B220 + cells from PP or CP. Solid line: CCR9 expression or CCL27 binding, grey histogram: human IgG Fc or isotype control. ( c , d ) Induction of CCR9 and CCR10 on IgA + cells by GALT-DCs. CD11c + cells were isolated from PP and CP of mice injected with B16 melanoma cells secreting Flt3L. Splenic naive B cells were cultured in the presence of antibody to IgM alone or with CP-derived DCs (CP-DC) or PP-derived DCs (PP-DC). After 4 days, B cells were analysed for CCR9 expression and CCL27 binding. ( c ) Each symbol represents an individual mouse, and horizontal bars indicate the mean. ( d ) Representative dot blots gated on B220 + cells are shown. Statistical analyses were performed with the Student’s t -test. * P <0.05. ** P <0.005, NS, not significant. Full size image Dendritic cells (DCs) residing in Peyer’s patches instruct B cells to secrete microbe-specific IgA [31] , and induce CCR9 expression on IgA-secreting cells [32] . Therefore, we analysed whether DCs in the caecal patch induce CCR10 expression on B cells ( Fig. 6c,d ). CD11c + DCs were isolated from Peyer’s patches and caecal patches of mice treated with FMS-like tyrosine kinase 3 ligand (Flt3L) and cultured with splenic naive B cells. Peyer’s patch-derived and caecal patch-derived DCs induced expression of CCR9 on B cells. In contrast, Peyer’s patch-derived DCs failed to induce CCR10 expression on cocultured B cells. However, B cells cocultured with caecal patch-derived DCs expressed increased levels of CCR10. Thus, DCs residing in the caecal patch were able to induce CCR10 expression. Increased colonic lymphoid clusters without caecal patch ILFs are sites of generation of IgA-secreting cells with differential mechanisms to those from Peyer’s patches [26] . In the absence of CCR10, SILTs including ILFs have been reported to enlarge and increase in number, which contributed to the maintenance of a normal number of IgA-secreting cells in the intestine of Ccr10 −/− mice [17] . Therefore, we measured the number of SILTs in the large intestine of appendectomized mice by whole-mount staining of B220 + cells at 8 weeks after conventionalization ( Fig. 7 ). The number of SILTs in the small intestine did not alter in appendectomized mice. In contrast, there were more SILTs in the large intestine of appendectomized mice than that of sham-operated mice. In addition, the size of each SILT was slightly larger in the large intestine of appendectomized mice. Thus, normalization of colonic IgA-secreting cells at 8 weeks correlates with the increased and enlarged SILTs. 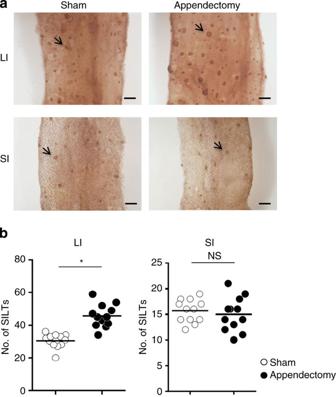Figure 7: Increased numbers of isolated lymphoid clusters in the colon of appendectomized mice. (a) SILTs were visualized based on B220+clusters (arrows) of whole-mount staining of intestines. Representative photos are shown. (b) Numbers of SILTs per surface of intestines (in a 25 mm square) are shown (12 mice analysed). Each symbol represents an individual mouse, and horizontal bars indicate the mean. Original magnification: × 7. Scale bars, 1 mm. SI: small intestine, LI: large intestine. Statistical analyses were performed with the Student’st-test. *P<0.05. NS, not significant. Figure 7: Increased numbers of isolated lymphoid clusters in the colon of appendectomized mice. ( a ) SILTs were visualized based on B220 + clusters (arrows) of whole-mount staining of intestines. Representative photos are shown. ( b ) Numbers of SILTs per surface of intestines (in a 25 mm square) are shown (12 mice analysed). Each symbol represents an individual mouse, and horizontal bars indicate the mean. Original magnification: × 7. Scale bars, 1 mm. SI: small intestine, LI: large intestine. Statistical analyses were performed with the Student’s t -test. * P <0.05. NS, not significant. Full size image In this study, we show that in the absence of the caecal patch, the number of IgA-secreting cells in the large intestine increased with markedly delayed kinetics after bacterial colonization. Subsequent analyses demonstrated that IgA-secreting plasmablasts migrate to the large and small intestines from the caecal patch, but plasmablasts in Peyer’s patches are mainly recruited to the small intestines. DCs in caecal patches, but not in Peyer’s patches, effectively induced expression of CCR10, which mediates recruitment of plasmablasts to both the small and large intestines. In line with the decreased number of IgA-secreting cells in the large intestine of appendectomized mice, the composition of microbiota in faeces altered compared with that of sham-operated mice at 4 weeks after conventionalization. We generated mice lacking the caecal patch using germ-free mice that developed normal adaptive immunity after colonization of microbiota. Appendectomy has been performed in mice reared in specific-pathogen-free condition [18] , [22] . However, in this condition, mice suffered from peritonitis due to extravasation of microbiota via surgical wound sites, and are therefore unsuitable for analysis of intestinal immune responses in the healthy state. In contrast, surgical operation of the appendix in germ-free mice did not cause inflammation because of an absence of microbiota, and the sutured wounds were almost completely closed within 1 week without any sign of inflammation. In addition, resection of the appendix did not cause dramatic reduction of the luminal space of the caecum as shown in Supplementary Fig. 2 . This enabled us to investigate the development of mucosal immunity in appendectomized mice after conventionalization. In accordance with the decreased number of IgA-secreting cells in the large intestine, the composition of faecal microbiota altered in appendectomized mice at 4 weeks after conventionalization. Therefore, as has been reported in the small intestine [7] , [8] , [12] , generation of IgA-secreting cells appears responsible for the maintenance of microbial homeostasis in the large intestine. Intriguingly, appendectomized mice at the early time point after conventionalization showed diverse patterns of microbial communities between individuals, whereas sham-operated mice contained microbiota that were highly homogeneous to each other. Thus, colonic secretory IgA contributes to shaping the microbial patterns characteristic of mice. IgAs in the small and large intestines have been reported to possess differential repertoires [15] . The differential diversities are thought to occur before plasma cell recruitment to the small and large intestines [15] . However, the events that govern the generation of distinct specificities of IgA remain unknown. The present study provides evidence that the caecal patch is the major site for the generation of plasmablasts migrating to both the small and large intestines, whereas Peyer’s patches are areas that generate plasmablasts that show preferential migration to the small intestine. Secretory IgA, which has differential diversities between the small and large intestines, has been shown to control gut microbiota [5] , [7] , [8] , [9] , [12] . As has been reported in the human intestine [33] , the caecum showed a similar pattern of bacterial composition to the large intestine. Thus, it is supposed that IgA generated in the caecal patch, which is exposed to the large intestine-types of microbiota, controls microbiota composition in the large intestine. However, at 8 weeks after conventionalization, microbiota composition was normalized in the large intestine of mice with appendectomy. Therefore, IgA generated in lymphoid tissues other than the caecal patch also contributes to the maintenance of microbiota homeostasis. Indeed, colonic SILTs including ILFs increased in mice with appendectomy. The chemokine receptors CCR9 and CCR10 have been shown to mediate the migration of IgA-secreting plasmablasts to the intestine. CCR9 is responsible for the homing to the small intestine [16] , whereas CCR10 contributes to the migration to both the small and large intestines [17] , [34] , [35] . IgA + cells in the caecal patch expressed higher levels of CCR9 and CCR10 than the cells in Peyer’s patches. Therefore, the higher expression of CCR10 on IgA-secreting cells generated in the caecal patch might be responsible for the preferential migration to the large intestine compared with cells instructed in Peyer’s patches. In accordance with the finding that DCs residing in Peyer’s patches induce generation of IgA-secreting cells and expression of CCR9 (ref. 32 ), DCs residing in the caecal patch induced enhanced levels of CCR10. Thus, IgA-secreting cells generated in the caecal patch might be programmed to migrate to the large intestine with enhanced CCR10 expression. CD11c + DCs residing in Peyer’s patch and the caecal patch showed differential activity in terms of CCR10 induction on IgA + cells. It would be an interesting future study to analyse the mechanisms of the differential properties of DCs residing in Peyer’s patch and the caecal patch. In contrast to the decreased number of IgA-secreting cells observed in the large intestine of appendectomized mice, the number of CD4 + T cells producing IFN-γ, IL-17 or IL-10 in the small and large intestines did not change. In this regard, several unique subsets of intestinal DCs that instruct development of Th1, Th17 or regulatory T cells have been identified [36] . These DCs reside in the lamina propria to sample luminal antigens, and migrate to mesenteric lymph nodes, where they induce effector and regulatory CD4 + T cells [37] , [38] , [39] . Thus, unlike IgA-secreting cells, development of helper and regulatory T cells are mediated by DCs that reside in the lamina propria. Therefore, the absence of the caecal patch did not affect T-cell development in the intestine. ILF has been shown to contribute to T-cell-independent IgA synthesis, the mechanism of which is different from that observed in Peyer’s patches [26] . In addition, ILFs have been shown to increase in number in the small and large intestines of mice lacking CCR10, which show normal numbers of IgA-secreting cells in the intestine [17] . Enlarged ILFs are considered to serve to compensate for the defective recruitment of Ccr10 −/− IgA-secreting cells to the intestine. Similarly to Ccr10 −/− mice, the number and size of ILFs in the large intestine increased in appendectomized mice in the current study. However, unlike Ccr10 −/− mice, which showed increased and enlarged SILTs in the small intestine, SILTs did not increase in the small intestine of mice with appendectomy after bacterial colonization. In this regard, CCR10 + IgA + cells generated in the colonic SILTs might be able to migrate to both the small and large intestine in our study. However, in the absence of CCR10, IgA + cells generated in the enlarged colonic SILTs were impaired in the migration to the small intestine and therefore SILTs in the small intestine might be enlarged in Ccr10 −/− mice. Collectively, our results demonstrate that a lymphoid organ in the appendix is a major tissue generating IgA + cells migrating to the large intestine. Peyer’s patches and the caecal patch have distinct properties in terms of induction of IgA + cells with differential migratory directions. This might correlate with the distinct functions of secretory IgAs in the small and large intestines. The precise characterization of IgA generated in Peyer’s patches and the caecal patch will reveal how differential IgA repertoires between the small and large intestines are generated in the future. Mice C57BL/6J mice and CD45.1 congenic mice of the C57BL/6 background (6–8-week old) were purchased from Japan SLC and Sankyo Laboratories Japan, respectively. ALY/NscJcl- aly ( aly/aly ) and ICR mice were from CLEA Japan. Kaede-transgenic mice [29] were kindly provided by Dr Michio Tomura (Kyoto University). These mice were kept under specific-pathogen-free conditions at the Experimental Animal Facility, Graduate School of Medicine, Osaka University. Germ-free (IQI/Jic[Gf] ICR) mice were from CLEA Japan and maintained under germ-free conditions. Tcrb −/− Tcrd −/− (refs 40 , 41 ) and Rorc ( gt ) gfp/gfp mice [42] of the C57BL/6 background were from Jackson Laboratory, and maintained at the Experimental Animal Facility, Institute of Medical Science, The University of Tokyo. Both male and female mice were used for the all experiments. All animal experiments were performed in accordance with the guidelines of Osaka University Animal Experiment and the Animal Care and Use Committee, The University of Tokyo. Antibodies FITC anti-IgM (1B4B1) and Phycoerythrin (PE) anti-IgA (11-44-2) mAbs were purchased from Southern Biotech. Pacific Blue anti-CD45R/B220 (RA3-6B2), FITC anti-CD45R/B220 (RA3-6B2), unlabelled anti-CD16/32 (2.4G2), biotin anti-IgA (C10-1), FITC anti-IgA (C10-3), APC rat IgG 2a isotype, APC anti-CD138/Syndecan-1 (281-2) and PE anti-CD11c (HL3) mAbs were from BD Biosciences. PerCP/Cy5.5 anti-CD4 (GK1.5), PE anti-IL-10 (JES5-16E3), Alexa Fluor 647 anti-IL-17A (TC11-18H10.1), FITC anti-IFN-γ (XMG1.2), APC/Cy7 anti-CD45R/B220 (RA3-6B2), Pacific Blue anti-CD45.2 (clone 104), Pacific Blue anti-CD11b (M1/70), Alexa Fluor 647 anti-mouse CCR9 (CW-1.2) mAbs and Alexa Fluor 647 mouse IgG 2a were from Biolegend. Human CCL27-Fc and control-Fc chimera proteins were as described previously [34] . Briefly, 293T cells were transfected with the CCL27-Fc and control-Fc expression vectors using Lipofectamine 2000 (Invitrogen). The culture supernatants containing these chimera proteins were collected and used for the experiments. Quantitative real-time PCR Total RNA was extracted with TRIzol reagent (Life Technologies). After treated with RQ1 DNase I (Promega), total RNA was reverse transcribed using M-MLV reverse transcriptase (Promega) and random primers (Toyobo). Complementary DNA was analysed by qPCR using GoTaq qPCR Master Mix (Promega) and an ABI 7300 system (Applied Biosystems). All values were normalized against the amount of glyceraldhyde-3-phosphate dehydrogenase (GAPDH) in each sample. Amplification conditions were: 50 °C (2 min), 95 °C (10 min) and 40 cycles of 95 °C (15 s) and 60 °C (60 s). The following primer sets were used: Gapdh , 5′-CCTCGTCCCGTAGACAAAATG-3′ and 5′-TCTCCACTTTGCCACTGCAA-3′; Tnfsf13 , 5′-AGACATTGTACGAGTCTGGGA-3′ and 5′-TCCCTTGTCCTTCCCGAGATA-3′; Tnfsf13c 5′-ATAGTGGTGAGGCAAACAGGC-3′ and 5′-CGTCCCCAAAGACGTGTACTT-3′; Aicda , 5′-AACCAGACAACTTCGGCGCAT-3′ and 5′-TCATCACGTGTGACATTCCAG-3′. Immunohistological staining Collected tissues were fixed with 4% paraformaldehyde for 1 h at 4 °C. After washing, tissues were incubated in a 30% sucrose solution overnight at 4 °C, and embedded in OCT compound (Sakura Finetech). Frozen sections of lymphoid tissues (10 μm) were blocked with PBS containing 0.5% Triton X-100 (PBS-T) and 3% bovine serum albumin (BSA), and incubated with APC anti-CD11c (5 μg ml −1 ), FITC anti-CD45R/B220(5 μg ml −1 ) and biotin anti-CD4 mAbs (5 μg ml −1 ), followed by streptavidin-Alexa Fluor 568 (Life Technologies) (2 μg ml −1 ). Alternatively, frozen sections were incubated with FITC anti-IgA (5 μg ml −1 ).The sections were incubated with DAPI (Vector Laboratories), and analysed using a confocal microscope (FV1000-D; Olympus). Surgical procedure In appendectomized groups, germ-free mice underwent incision (2 cm in length) on the abdomen under anaesthesia, and the appendix was gently pulled out, ligated with 5-0 Polydioxanone Suture (Ethicon) at the border between the appendix and caecum, and resected in a vinyl isolator. This procedure ensured complete removal of appendix lymphoid tissues and minimized contamination. The caecal stump was irrigated with PBS and the wound was closed. In sham-operated groups, germ-free mice underwent incision of the abdomen and the wound was closed without further treatment. After surgery, mice were maintained under germ-free condition for 1 week. Mice were then transferred to specific-pathogen-free conditions and kept for 2, 4 or 8 weeks (see also Supplementary Figs 2 and 5a ). The appendectomized mice were kept separately from the sham-operated mice. Each group was housed in one cage. Isolation of lymphocytes To prepare lymphocytes from Peyer’s patches and caecal patches, tissues were gently squeezed between glass slides, and the cells were passed through 40 μm nylon meshes. Intestinal lamina propria lymphocytes were prepared as described previously [43] . Briefly, the small and large intestines were opened, washed to remove faecal content, shaken in HBSS containing 5 mM EDTA for 20 min at 37 °C and cut into small pieces, and incubated with RPMI 1640 containing 4% fetal bovine serum (FBS), 1 mg ml −1 collagenase D (Roche), 0.5 mg ml −1 dispase (Invitrogen) and 40 μg ml −1 DNase I (Roche) for 1 h at 37 °C in a shaking water bath. The digested tissues were subjected to Percoll density-gradient (40%/70%) centrifugation. The lamina propria lymphocytes were collected at the interface of the Percoll gradient. Intracellular cytokine staining Intracellular expression of IFN-γ, IL-17 and IL-10 in CD4 + T cells was analysed using a Cytofix/Cytoperm Kit Plus (BD Biosciences) according to the manufacturer’s instructions. Briefly, lymphocytes obtained from the intestinal lamina propria were incubated with 50 ng ml −1 of phorbol myristate acetate (Sigma), 5 μM of calcium ionophore A23187 (Sigma) and Golgistop at 37 °C for 4 h. Cells were incubated with PerCP/Cy5.5 anti-CD4 mAb (2 μg ml −1 ). After Fix/Perm treatment for 20 min, intracellular cytokine staining was performed with PE anti-IL-10 (2 μg ml −1 ), FITC anti-IFN-γ (5 μg ml −1 ) and Alexa Fluor 647 anti-IL-17A(5 μg ml −1 ) mAbs for 20 min. Flow cytometry Cells were treated with anti-CD16/32 mAb (10 μg ml −1 ) in PBS containing 2% FBS to block nonspecific binding, and incubated with the indicated mAbs. Samples were incubated with 7-amino-actinomycinD (1 μg ml −1 ) to exclude dead cells before analyses. Flow cytometry was performed using a FACSCanto II flow cytometer (BD Biosciences) with FlowJo software (Tree Star). To measure the absolute number of CD4 + T cell subsets and surface IgA + cells in the intestine, total number of cells isolated from tissues was counted, and then proportion of each cell population was determined by flow cytometry. The number of CD4 + T cell subsets and surface IgA + cells was calculated as ‘total cell number’ × ‘percentage in flow cytometry’. For cell isolation, cells were sorted using FACSAria (BD Biosciences). Measurement of IgA To prepare faecal samples, faeces were homogenized in PBS (1 mg faeces in 10 ml PBS), and subjected to stepwise centrifugation with increasing force (400 g for 5 min, 8,000 g for 10 min and 19,000 g for 10 min) to remove debris. To prepare mononuclear cells in tissues, Peyer’s patches and the caecal patch were shaken for 20 min at 37 °C in HBSS containing 5 mM EDTA to remove epithelial cells. The tissues were digested with 1 mg ml −1 Collagenase D (Roche Diagnostics) and applied to a discontinuous 40 and 70% Percoll density gradient (GE Healthcare). The mononuclear cells were then cultured for 3 days and the culture supernatants were collected. IgA levels in the faeces, sera and culture supernatants were determined by a mouse IgA ELISA quantitation kit (Bethyl Laboratories). Optical densities were determined at a wavelength of 450 nm with a reference wavelength of 570 nm. Extraction of bacterial DNA from faeces Faeces were collected in collection tubes containing RNA later (Ambion). After weighing, RNA later was added to make a 10-fold diluted faecal homogenate. The homogenate (200 μl) was washed twice with 1 ml PBS. Glass beads (0.3 g; diameter, 0.1 mm; (BioSpec Products), 300 μl Tris-SDS solution and 500 μl TE-saturated phenol were added to the suspension, and the mixture was vortexed vigorously for 30 s using a FastPrep-24 (MP Biomedicals) at 5.0 power level for 30 s. After centrifugation at 20,000 g for 5 min at 4 °C, 400 μl of the supernatant was collected. Subsequently, phenol–chloroform extraction was performed and 250 μl of the supernatant was subjected to isopropanol precipitation. Finally, the DNA was suspended in 200 μl of TE buffer and stored at −20 °C. Determination of microbiota by 16S rRNA pyrosequencing PCR was performed using a primer set (784F: 5′-AGGATTAGATACCCTGGTA-3′ and 1061R: 5′-CRRCACGAGCTGACGAC-3′) targeting the V5–V6 region of the 16S rRNA genes [44] . To amplify the targeted region, 1 μl of extracted DNA served as the template in 50 μl reactions using KAPA HiFi HS Ready Mix (KAPA Biosystems). PCR conditions were 95 °C for 3 min, 25 cycles at 98 °C for 20 s, 60 °C for 15 s and 72 °C for 15 s. Two 100-μl three-cycle reconditioning PCR reactions were performed per sample to eliminate heteroduplexes, with 10 μl aliquots of the initial PCR product mixture as the template and other PCR conditions unchanged. Products of the two reconditioning PCR reactions per sample were combined and purified using DNA clean and Concentrator-5 (Zymo Research). Amplified PCR products were used as a template for pyrosequencing with the GS Junior platform (Roche). Pyrosequencing was performed by following the manufacturer’s instruction using MID tags. Raw sequences were demultiplexed and quality-trimmed using the QIIME pipeline [45] with default parameters. The trimmed sequences were denoised using AmpliconNoise version 1.2.7 (ref. 46 ). USEARCH version 6.0.203 (ref. 47 ) was employed to remove chimaera sequences using the SILVA 111 database [48] as a reference. The processed sequences were then clustered into OTU defined at 97% similarity cutoff using UCLUST version 1.2.22q (ref. 47 ). Representative sequences for each OTU were classified taxonomically using RDP Classifier version 2.2 (ref. 49 ) with the SILVA 111 database. Rarefaction curves and UniFrac (ref. 50 ) distance matrixes were generated using the QIIME tool. The relative abundance was represented as the ratio of the bacterial group to the whole microbiota. Photoconversion Kaede bone marrow chimeric mice were generated by intravenous injection of Kaede-labelled bone marrow cells (2 × 10 6 ) into 9.5-Gy-irradiated wild-type C57BL/6 mice. Mice were allowed to reconstitute for at least 6 weeks before experimental procedures. For photoconversion, mice were anaesthetized with isoflurane, and a skin incision was made in the abdominal skin to expose Peyer’s patches and caecal patches. The surrounding tissue was covered with aluminium foil to prevent unnecessary exposure, and the tissues were exposed to violet light (200 mW cm −2 ) with a 436-nm g-line band-pass filter with spot UV curing equipment (SP500; Usio) for 5 min. The abdominal wall was closed by 9-mm Autoclips (Clay Adams). Adoptive transfer experiments B220 + cells were positively separated using the MACS separation system (Miltenyi Biotec) from Peyer’s patches and caecal patches of CD45.2 mice. Sorted cells (1 × 10 6 ) were intravenously injected into C57BL/6 CD45.1 recipients through the retro-orbital plexus. Seven days after injection, the lymphocytes were isolated from the small and large intestinal lamina propria and analysed using a flow cytometer. B-cell activation and coculture with GALT-DCs To prepare GALT-DCs, C57BL/6 mice were injected s.c. with B16 cells secreting Flt3L as described [51] . After 14 days of the injection, Peyer’s patches and caecal patches were isolated and digested with RPMI1640 containing 4% FBS, 1 mg ml −1 collagenase D (Roche Diagnostics) and 40 μg ml −1 DNase I (Roche Diagnostics) for 30 min at 37 °C. Cells were spun through a 17.5% Accudenz solution (Accurate Chemical & Scientific Corporation). Obtained cells were incubated with PE anti-CD11c (2 μg ml −1 ) and subjected to cell sorting (FACSAria). CD11c + cells with >95% purity were used for the experiments. Naive B cells were purified from the spleen by negative selection using anti-CD43 microbeads (Miltenyi Biotec). Purified naive B cells (5 × 10 5 ) were cultured in the presence of 10 μg ml −1 anti-mouse IgM F(ab′) 2 (Jackson ImmunoResearch) alone or with equivalent numbers of Peyer’s patch-derived or caecal patch-derived DCs for 4 days [32] . Whole-mount microscopic analysis Whole-mount microscopic analysis was performed as described previously [52] . Briefly, the small and large intestines were removed intact, opened along the mesenteric border, flushed with PBS and mounted in 8-cm segments from proximal to distal. Samples were then incubated in Hank’s balanced salt solution containing 5 mM EDTA at 37 °C with shaking for 10 min to remove epithelial cells, followed by washing with cold PBS. Samples were fixed in 4% paraformaldehyde for 1 h, washed with PBS-T and incubated with 1% H 2 O 2 in methanol to block endogenous peroxidases. Samples were then incubated with PBS-T containing 3% BSA for 30 min with shaking, and incubated with anti-CD45R/B220 mAb (5 μg ml −1 ) overnight at 4 °C, followed by HRP-conjugated F(ab′) 2 goat anti-rat IgG Ab (Jackson ImmunoResearch) (1 μg ml −1 ) at room temperature for 1 h. Signals were developed with Metal Enhanced DAB substrate (Thermo Scientific). Samples were analysed using an Olympus stereo microscope SZX-12. Statistical analysis Differences between control and experimental groups were evaluated using the Student’s t -test. A P value <0.05 was considered statistically significant. Data are presented as mean±s.d. Mann–Whitney U /Wilcoxon rank sum tests were conducted to assess significant differences in relative abundance of specific OTU obtained by microbiota analysis. For multivariate analyses of data, principal component analysis was used to visualize data sets by statistical programming language R 2.1.5. Between-class analysis and principal coordinate analysis were calculated using the R package ‘ade4’. In the UniFrac analysis, ANOSIM was calculated using R package ‘vegan’. How to cite this article: Masahata, K. et al. Generation of colonic IgA-secreting cells in the caecal patch. Nat. Commun. 5:3704 doi: 10.1038/ncomms4704 (2014).